Frequent mutations in chromatin-remodelling genes in pulmonary carcinoids Pulmonary carcinoids are rare neuroendocrine tumours of the lung. The molecular alterations underlying the pathogenesis of these tumours have not been systematically studied so far. Here we perform gene copy number analysis ( n =54), genome/exome ( n =44) and transcriptome ( n =69) sequencing of pulmonary carcinoids and observe frequent mutations in chromatin-remodelling genes. Covalent histone modifiers and subunits of the SWI/SNF complex are mutated in 40 and 22.2% of the cases, respectively, with MEN1 , PSIP1 and ARID1A being recurrently affected. In contrast to small-cell lung cancer and large-cell neuroendocrine lung tumours, TP53 and RB1 mutations are rare events, suggesting that pulmonary carcinoids are not early progenitor lesions of the highly aggressive lung neuroendocrine tumours but arise through independent cellular mechanisms. These data also suggest that inactivation of chromatin-remodelling genes is sufficient to drive transformation in pulmonary carcinoids. Pulmonary carcinoids are neuroendocrine tumours that account for about 2% of pulmonary neoplasms. On the basis of the WHO classification of 2004, carcinoids can be subdivided into typical or atypical, the latter ones being very rare (about 0.2%) [1] . Most carcinoids can be cured by surgery; however, inoperable tumours are mostly insensitive to chemo- and radiation therapies [1] . Apart from few low-frequency alterations, such as mutations in MEN1 (ref. 1 ), comprehensive genome analyses of this tumour type have so far been lacking. Here we conduct integrated genome analyses [2] on data from chromosomal gene copy number of 54 tumours, genome and exome sequencing of 29 and 15 tumour-normal pairs, respectively, as well as transcriptome sequencing of 69 tumours. Chromatin-remodelling is the most frequently mutated pathway in pulmonary carcinoids; the genes MEN1 , PSIP1 and ARID1A were recurrently affected by mutations. Specifically, covalent histone modifiers and subunits of the SWI/SNF (SWich/Sucrose NonFermentable) complex are mutated in 40 and 22.2% of the cases, respectively. By contrast, mutations of TP53 and RB1 are only found in 2 out of 45 cases, suggesting that these genes are not main drivers in pulmonary carcinoids. 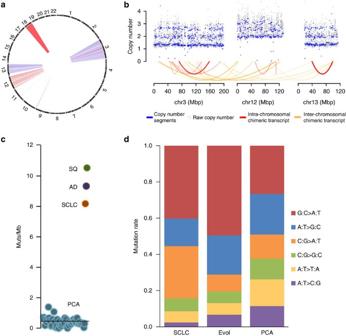Figure 1: Genomic characterization of pulmonary carcinoids. (a) CIRCOS plot of the chromothripsis case. The outer ring shows chromosomes arranged end to end. Somatic copy number alterations (gains in red and losses in blue) detected by 6.0 SNP arrays are depicted in the inside ring. (b) Copy numbers and chimeric transcripts of affected chromosomes. Segmented copy number states (blue points) are shown together with raw copy number data averaged over 50 adjacent probes (grey points). To show the different levels of strength for the identified chimeric transcripts, all curves are scaled according to the sequencing coverage at the fusion point. (c) Mutation frequency detected by genome and exome sequencing in pulmonary carcinoids (PCA). Each blue dot represents the number of mutations (muts) per Mb in one pulmonary carcinoid sample. Average frequencies are also shown for adenocarcinomas (AD), squamous (SQ) and small-cell lung cancer (SCLC) based on previous studies2,4,5. (d) Comparison of context-independent transversion and transition rates (an overall strand symmetry is assumed) between rates derived from molecular evolution (evol)36, from a previous SCLC sequencing study2and from the PCA genome and exome sequencing. All rates are scaled such that their overall sum is 1. In total, we generated genome/exome sequencing data for 44 independent tumour-normal pairs, and for most of them, also RNAseq ( n =39, 69 in total) and SNP 6.0 ( n =29, 54 in total) data ( Supplementary Table 1 ). Although no significant focal copy number alterations were observed across the tumours analysed, we detected a copy number pattern compatible with chromothripsis [3] in a stage-III atypical carcinoid of a former smoker ( Fig. 1a ; Supplementary Fig. 1 ). The intensely clustered genomic structural alterations found in this sample were restricted to chromosomes 3, 12 and 13, and led to the expression of several chimeric transcripts ( Fig. 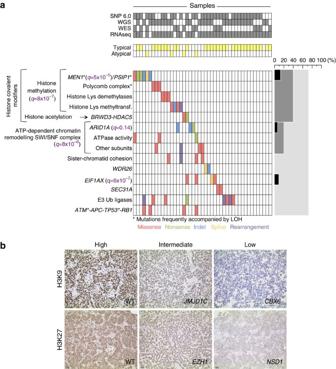Figure 2: Significant affected genes and pathways in pulmonary carcinoids. (a) Significantly mutated genes and pathways identified by genome (n=29), exome (n=15) and transcriptome (n=69) sequencing. The percentage of pulmonary carcinoids with a specific gene or pathway mutated is noted at the right side. Theq-values of the significantly mutated genes and pathways are shown in brackets (see Methods section). Samples are displayed as columns and arranged to emphasize mutually exclusive mutations. (b) Methylation levels of H3K9me3 and H3K27me3 in pulmonary carcinoids. Representative pictures of different degrees of methylation (high, intermediate and low) for some of the samples summarized inTable 1. The mutated gene is shown in italics at the bottom right part of the correspondent picture. Wild-type samples are denoted by WT. 1b ; Supplementary Table 2 ). Some of these chimeric transcripts affected genes involved in chromatin-remodelling processes, including out-of-frame fusion transcripts disrupting the genes ARID2 , SETD1B and STAG1. Through the analyses of genome and exome sequencing data, we detected 529 non-synonymous mutations in 494 genes, which translates to a mean somatic mutation rate of 0.4 mutations per megabase (Mb) ( Fig. 1c ; Supplementary Data 1 ), which is much lower than the rate observed in other lung tumours ( Fig. 1c ) [2] , [4] , [5] . As expected, and in contrast to small-cell lung cancer (SCLC), no smoking-related mutation signature was observed in the mutation pattern of pulmonary carcinoids ( Fig. 1d ). Figure 1: Genomic characterization of pulmonary carcinoids. ( a ) CIRCOS plot of the chromothripsis case. The outer ring shows chromosomes arranged end to end. Somatic copy number alterations (gains in red and losses in blue) detected by 6.0 SNP arrays are depicted in the inside ring. ( b ) Copy numbers and chimeric transcripts of affected chromosomes. Segmented copy number states (blue points) are shown together with raw copy number data averaged over 50 adjacent probes (grey points). To show the different levels of strength for the identified chimeric transcripts, all curves are scaled according to the sequencing coverage at the fusion point. ( c ) Mutation frequency detected by genome and exome sequencing in pulmonary carcinoids (PCA). Each blue dot represents the number of mutations (muts) per Mb in one pulmonary carcinoid sample. Average frequencies are also shown for adenocarcinomas (AD), squamous (SQ) and small-cell lung cancer (SCLC) based on previous studies [2] , [4] , [5] . ( d ) Comparison of context-independent transversion and transition rates (an overall strand symmetry is assumed) between rates derived from molecular evolution (evol) [36] , from a previous SCLC sequencing study [2] and from the PCA genome and exome sequencing. All rates are scaled such that their overall sum is 1. Full size image We identified MEN1 , ARID1A and EIF1AX as significantly mutated genes [2] ( q- value <0.2, see Methods section) ( Fig. 2a ; Supplementary Tables 1 and 3 ; Supplementary Data 1 ). MEN1 and ARID1A play important roles in chromatin-remodelling processes. The tumour suppressor MEN1 physically interacts with MLL and MLL2 to induce gene transcription [6] . Specifically, MEN1 is a molecular adaptor that physically links MLL with the chromatin-associated protein PSIP1, an interaction that is required for MLL/MEN1-dependent functions [7] . MEN1 also acts as a transcriptional repressor through the interaction with SUV39H1 [8] . We observed mutually exclusive frame-shift and truncating mutations in MEN1 and PSIP1 in six cases (13.3%), which were almost all accompanied by loss of heterozygosity ( Supplementary Fig. 2 ). We also detected mutations in histone methyltransferases ( SETD1B , SETDB1 and NSD1 ) and demethylases ( KDM4A , PHF8 and JMJD1C ), as well as in the following members of the Polycomb complex [9] ( Supplementary Tables 1 and 2 ; Supplementary Data 1 ): CBX6 , which belongs to the Polycomb repressive complex 1 (PRC1); EZH1, which is part of the PCR2; and YY1 , a member of the PHO repressive complex 1 that recruits PRC1 and PRC2. CBX6 and EZH1 mutations were also accompanied by loss of heterozygosity ( Supplementary Fig. 2 ). In addition, we also detected mutations in the histone modifiers BRWD3 and HDAC5 in one sample each. In total, 40% of the cases carried mutually exclusive mutations in genes that are involved in covalent histone modifications ( q -value=8 × 10 −7 , see Methods section) ( Fig. 2a ; Supplementary Table 4 ). To evaluate the impact of these mutations on histone methylation, we compared the levels of the H3K9me3 and H3K27me3 on seven mutated and six wild-type samples, and observed a trend towards lower methylation in the mutated cases ( Fig. 2b ; Table 1 ). Figure 2: Significant affected genes and pathways in pulmonary carcinoids. ( a ) Significantly mutated genes and pathways identified by genome ( n =29), exome ( n =15) and transcriptome ( n =69) sequencing. The percentage of pulmonary carcinoids with a specific gene or pathway mutated is noted at the right side. The q -values of the significantly mutated genes and pathways are shown in brackets (see Methods section). Samples are displayed as columns and arranged to emphasize mutually exclusive mutations. ( b ) Methylation levels of H3K9me3 and H3K27me3 in pulmonary carcinoids. Representative pictures of different degrees of methylation (high, intermediate and low) for some of the samples summarized in Table 1 . The mutated gene is shown in italics at the bottom right part of the correspondent picture. Wild-type samples are denoted by WT. Full size image Table 1 Overview of samples annotated for mutations in genes involved in histone methylation and correspondent levels of H3K9me3 and H3K27me3 detected by immunohistochemistry. Full size table Truncating and frame-shift mutations in ARID1A were detected in three cases (6.7%). ARID1A is one of the two mutually exclusive ARID1 subunits, believed to provide specificity to the ATP-dependent SWI/SNF chromatin-remodelling complex [10] , [11] . Truncating mutations of this gene have been reported at high frequency in several primary human cancers [12] . In total, members of this complex were mutated in mutually exclusive fashion in 22.2% of the specimens ( q -value=8 × 10 −8 , see Methods section) ( Fig. 2a ; Supplementary Table 4 ). Among them were the core subunits SMARCA1 , SMARCA2 and SMARCA4 , which carry the ATPase activity of the complex, as well as the subunits ARID2, SMARCC2 , SMARCB1 and BCL11A ( Fig. 2a ; Supplementary Tables 1 and 2 ; Supplementary Data 1 ) [13] , [14] . Another recurrently affected pathway was sister-chromatid cohesion during cell cycle progression with the following genes mutated ( Fig. 2a ; Supplementary Tables 1 and 2 ; Supplementary Data 1 ; Supplementary Fig. 3 ): the cohesin subunit STAG1 (ref. 15 ), the cohesin loader NIPBL [16] ; the ribonuclease and microRNA processor DICER , necessary for centromere establishment [17] ; and ERCC6L, involved in sister-chromatid separation [18] . In addition, although only few chimeric transcripts were detected in the 69 transcriptomes analysed ( Supplementary Table 5 ), we found one sample harbouring an inactivating chimeric transcript, leading to the loss of the mediator complex gene MED24 ( Supplementary Fig. 4 ) that interacts both physically and functionally with cohesin and NIPBL to regulate gene expression [19] . In summary, we detected mutations in chromatin-remodelling genes in 23 (51.1%) of the samples analysed. The specific role of histone modifiers in the development of pulmonary carcinoids was confirmed by the lack of significance of these pathways in SCLC [2] ( Supplementary Table 4 ). This was further supported by a gene expression analysis including 49 lung adenocarcinomas (unpublished data), 43 SCLC [2] , [20] and the 69 pulmonary carcinoids included in this study ( Supplementary Data 2 ). Consensus k-means clustering revealed that although both SCLC and pulmonary carcinoids are lung neuroendocrine tumours, both tumour types as well as adenocarcinomas formed statistically significant separate clusters ( Fig. 3a ). In support of this notion, we recently reported that the early alterations in SCLC universally affect TP53 and RB1 [2] , whereas in this study these genes were only mutated in two samples ( Fig. 2a ; Supplementary Table 1 ; Supplementary Data 1 ). Moreover, when examining up- and downregulated pathways in SCLC versus pulmonary carcinoids by gene set enrichment analysis [21] , we found that in line with the pattern of mutations, the RB1 pathway was statistically significantly altered in SCLC ( q -value=5 × 10 −4 , see Methods section) but not in pulmonary carcinoids ( Fig. 3b ; Supplementary Table 6 ). 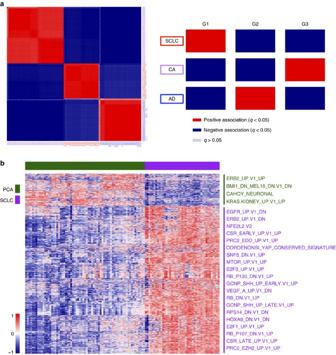Figure 3: Expression data analysis of pulmonary carcinois based on RNAseq data. (a) Consensus k-means clustering32,33using RNAseq expression data of 49 adenocarcinomas (AD, in blue), 43 small-cell lung cancer (SCLC, in red) and 69 pulmonary carcinoids (PCA, in purple) identified three groups using the clustering module from GenePattern31and consensus CDF32,33(left panel). The significance of the clustering was evaluated by using SigClust34with aP<0.0001. Fisher’s exact test35was used to check associations between the clusters and the histological subtypes (right panel). (b) Gene set enrichment analysis21for SCLC versus PCA using RNAseq expression data. Low gene expression is indicated in blue and high expression, in red. On the right side are given the altered pathways in PCA (green) and SCLC (purple). Figure 3: Expression data analysis of pulmonary carcinois based on RNAseq data. ( a ) Consensus k-means clustering [32] , [33] using RNAseq expression data of 49 adenocarcinomas (AD, in blue), 43 small-cell lung cancer (SCLC, in red) and 69 pulmonary carcinoids (PCA, in purple) identified three groups using the clustering module from GenePattern [31] and consensus CDF [32] , [33] (left panel). The significance of the clustering was evaluated by using SigClust [34] with a P <0.0001. Fisher’s exact test [35] was used to check associations between the clusters and the histological subtypes (right panel). ( b ) Gene set enrichment analysis [21] for SCLC versus PCA using RNAseq expression data. Low gene expression is indicated in blue and high expression, in red. On the right side are given the altered pathways in PCA (green) and SCLC (purple). Full size image Another statistically significant mutated gene was the eukaryotic translation initiation factor 1A ( EIF1AX ) mutated in four cases (8.9%). In addition, SEC31A, WDR26 and the E3 ubiquitin ligase HERC2 were mutated in two samples each. Further supporting a role of E3 ubiquitin ligases in the development of pulmonary carcinoids, we found mutations or rearrangements affecting these genes in 17.8% of the samples analysed ( Fig. 2a ; Supplementary Tables 1 and 7 ; Supplementary Data 1 ). All together, we have identified candidate driver genes in 73.3% of the cases. Of note, we did not observe any genetic segregation between typical or atypical carcinoids, neither between the expression clusters generated from the two subtypes, nor between these clusters and the mutated pathways ( Supplementary Fig. 5 ). However, it is worth mentioning that only nine atypical cases were included in this study. The spectrum of mutations found in the discovery cohort was further validated by transcriptome sequencing of an independent set of pulmonary carcinoid specimens ( Supplementary Tables 1 and 8 ). Owing to the fact that many nonsense and frame-shift mutations may result in nonsense-mediated decay [22] , [23] , the mutations detected by transcriptome sequencing were only missense. Owing to this bias, accurate mutation frequencies could not be inferred from these data. This study defines recurrently mutated sets of genes in pulmonary carcinoids. The fact that almost all of the reported genes were mutated in a mutually exclusive manner and affected a small set of cellular pathways defines these as the key pathways in this tumour type. Given the frequent mutations affecting the few signalling pathways described above and the almost universal absence of other cancer mutations, our findings support a model where pulmonary carcinoids are not early progenitor lesions of other neuroendocrine tumours, such as SCLC or large-cell neuroendocrine carcinoma, but arise through independent cellular mechanisms. More broadly, our data suggest that mutations in chromatin-remodelling genes, which in recent studies were found frequently mutated across multiple malignant tumours [24] , are sufficient to drive early steps in tumorigenesis in a precisely defined spectrum of required cellular pathways. Tumour specimens The study as well as written informed consent documents had been approved by the Institutional Review Board of the University of Cologne. Additional biospecimens for this study were obtained from the Victorian Cancer Biobank, Melbourne, Australia; the Vanderbilt-Ingram Cancer Center, Nashville, Tennessee, USA; and Roy Castle Lung Cancer Research Programme, The University of Liverpool Cancer Research Center, Liverpool, UK. The Institutional Review Board of each participating institution approved collection and use of all patient specimens in this study. Nucleic acid extraction and sample sequencing All samples in this study were reviewed by expert pathologists. Total RNA and DNA were obtained from fresh-frozen tumour and matched fresh-frozen normal tissue or blood. Tissue was frozen within 30 min after surgery and was stored at −80 °C. Blood was collected in tubes containing the anticoagulant EDTA and was stored at −80 °C. Total DNA and RNA were extracted from fresh-frozen lung tumour tissue containing more than 70% tumour cells. Depending on the size of the tissue, 15–30 sections, each 20 μm thick, were cut using a cryostat (Leica) at −20 °C. The matched normal sample obtained from frozen tissue was treated accordingly. DNA from sections and blood was extracted using the Puregene Extraction kit (Qiagen) according to the manufacturer’s instructions. DNA was eluted in 1 × TE buffer (Qiagen), diluted to a working concentration of 150 ng μl −1 and stored at −80 °C. For whole exome sequencing, we fragmented 1 μg of DNA with sonification technology (Bioruptor, diagenode, Liége, Belgium). The fragments were end repaired and adaptor ligated, including incorporation of sample index barcodes. After size selection, we subjected the library to an enrichment process with the SeqCap EZ Human Exome Library version 2.0 kit (Roche NimbleGen, Madison, WI, USA). The final libraries were sequenced with a paired-end 2 × 100 bp protocol. On average, 7 Gb of sequence were produced per normal, resulting in 30 × coverage of more than 80% of target sequences (44 Mb). For better sensitivity, tumours were sequenced with 12 Gb and 30 × coverage of more than 90% of target sequences. We filtered primary data according to signal purity with the Illumina Realtime Analysis software. Whole-genome sequencing was also performed using a read length of 2 × 100 bp for all samples. On average, 110 Gb of sequence were produced per sample, aiming a mean coverage of 30 × for both tumour and matched normal. RNAseq was performed on complementary DNA libraries prepared from PolyA+ RNA extracted from tumour cells using the Illumina TruSeq protocol for mRNA. The final libraries were sequenced with a paired-end 2 × 100 bp protocol aiming at 8.5 Gb per sample, resulting on a 30 × mean coverage of the annotated transcriptome. All the sequencing was carried on an Illumina HiSeq 2000 sequencing instrument (Illumina, San Diego, CA, USA). Sequence data processing and mutation detection Raw sequencing data are aligned to the most recent build of the human genome (NCBI build 37/hg19) using BWA (version: 0.5.9rc1) [25] and possible PCR duplicates are subsequently removed from the alignments. Somatic mutations were detected using our in-house-developed sequencing analysis pipeline. In brief, the mutation-calling algorithm incorporates parameters such as local copy number profiles, estimates of tumour purity and ploidy, local sequencing depth, as well as the global sequencing error into a statistical model with which the presence of a mutated allele in the tumour is determined. Next, the absence of this variant in the matched normal is assessed by demanding that the corresponding allelic fraction is compatible with the estimated background sequencing error in the normal. In addition, we demand that the allelic fractions between tumour and normal differ significantly. To finally remove artificial mutation calls, we apply a filter that is based on the forward–reverse bias of the sequencing reads. Further details of this approach are given in Peifer et al. [2] Genomic rearrangement reconstruction from paired-end data To reconstruct rearrangements from paired-end data, we refined our initial method [2] by adding breakpoint-spanning reads. Here, locations of encompassing read pairs are screened for further reads where only one pair aligns to the region and the other pair either does not align at all or is clipped by the aligner. These reads are then realigned using BLAT to a 1,000 bp region around the region defined by the encompassing reads. Rearrangements confirmed by at least one spanning read are finally reported. To filter for somatic rearrangements, we subtracted those regions where rearrangements are present in the matched normal and in all other sequenced normals within the project. Analysis of significantly mutated genes and pathways The analysis of significantly mutated genes is done in a way that both gene expression and the accumulation of synonymous mutations are considered to obtain robust assessments of frequently mutated, yet biologically relevant genes. To this end, the overall background mutation rate is determined first, from which the expected number of mutations for each gene is computed under the assumption of a purely random mutational process. This gene-specific expected number of mutations defines the underlying null model of our statistical test. To account for misspecifications, for example, due to a local variation of mutation rates, we also incorporated the synonymous to non-synonymous ratio into a combined statistical model to determine significantly mutated genes. Since mutation rates in non-expressed genes are often high than the genome-wide background rate [2] , [26] , genes that are having a median Fragments Per Kilobase of transcript per Million fragments mapped (FPKM) value <1 in our transcriptome sequencing data are removed prior testing. To account for multiple hypothesis testing, we are using the Benjamini–Hochberg approach [27] . Mutation data of the total of 44 samples, for which either whole-exome sequencing (WES) or whole-genome sequencing (WGS) was performed, were used for this analysis. In case of the pathway analysis, gene lists of the methylation and the SWI/SNF complex were obtained from recent publications [9] , [13] , [14] , [28] . To assess whether mutations in these pathways are significantly enriched, all genes of the pathway are grouped together as if they represent a ‘single gene’ and subsequently tested if the total number of mutation exceed mutational background of the entire pathway. To this end, the same method as described above was used. Mutation data of the total of 44 samples, for which either WES or WGS was performed, were used for this analysis. Analysis of chromosomal gene copy number data Hybridization of the Affymetrix SNP 6.0 arrays was carried out according to the manufacturers’ instructions and analysed as follows: raw signal intensities were processed by applying a log-linear model to determine allele-specific probe affinities and probe-specific background intensities. To calibrate the model, a Gauss–Newton approach was used and the resulting raw copy number profiles are segmented by applying the circular binary segmentation method [29] . Analysis of RNAseq data For the analysis of RNAseq data, we have developed a pipeline that affords accurate and efficient mapping and downstream analysis of transcribed genes in cancer samples (Lynnette Fernandez-Cuesta and Ruping Sun, personal communication). In brief, paired-end RNAseq reads were mapped onto hg19 using a sensitive gapped aligner, GSNAP [30] . Possible breakpoints were called by identifying individual reads showing split-mapping to distinct locations as well as clusters of discordant read pairs. Breakpoint assembly was performed to leverage information across reads anchored around potential breakpoints. Assembled contigs were aligned back to the reference genome to confirm bona fide fusion points. Dideoxy sequencing All non-synonymous mutations found in the genome/exome data were checked in RNAseq data when available. Genes recurrently mutated involved in pathways statistically significantly mutated, or interesting because of their presence in other lung neuroendocrine tumours, were selected for validation. One hundred and fifty eight mutations were considered for validation: 115 validated and 43 did not (validation rate 73%). Sequencing primer pairs were designed to enclose the putative mutation ( Supplementary Data 1 ), or to encompass the candidate rearrangement ( Supplementary Table 7 ) or chimeric transcript ( Supplementary Table 2 and 5 ). Sequencing was carried out using dideoxy-nucleotide chain termination (Sanger) sequencing, and electropherograms were analysed by visual inspection using four Peaks. Gene expression data analyses Unsupervised consensus clustering was applied to RNAseq data of 69 pulmonary carcinoids, 49 adenocarcinomas and 43 SCLC [2] , [20] samples. The 3,000 genes with highest variation across all samples were filtered out before performing consensus clustering. We used the clustering module from GenePattern [31] and the consensus CDF [32] , [33] . Significance was obtained by using SigClust [34] . Fisher’s exact test [35] was used to check for associations between clusters and histological subtypes. gene set enrichment analysis [21] were performed on 69 pulmonary carcinoids and 43 SCLC [2] , [20] samples; and the gene set oncogenic signatures were used. Accession codes: Whole genome sequence data, whole exome sequence data, transcriptome sequence data and affymetrix 6.0 (copy number) data have been deposited at the European Genome-phenome Archive under the accession code EGAS00001000650. How to cite this article: Fernandez-Cuesta, L. et al. Frequent mutations in chromatin-remodelling genes in pulmonary carcinoids. Nat. Commun. 5:3518 doi: 10.1038/ncomms4518 (2014).